SLC7A14 linked to autosomal recessive retinitis pigmentosa Retinitis pigmentosa (RP) is characterized by degeneration of the retinal photoreceptors and is the leading cause of inherited blindness worldwide. Although few genes are known to cause autosomal recessive RP (arRP), a large proportion of disease-causing genes remain to be revealed. Here we report the identification of SLC7A14 , a potential cationic transporter, as a novel gene linked to arRP. Using exome sequencing and direct screening of 248 unrelated patients with arRP, we find that mutations in the SLC7A14 gene account for 2% of cases of arRP. We further demonstrate that SLC7A14 is specifically expressed in the photoreceptor layer of the mammalian retina and its expression increases during postnatal retinal development. In zebrafish, downregulation of slc7a14 expression leads to an abnormal eye phenotype and defective light-induced locomotor response. Furthermore, targeted knockout of Slc7a14 in mice results in retinal degeneration with abnormal ERG response. This suggests that SLC7A14 has an important role in retinal development and visual function. Retinitis pigmentosa (RP) is a heterogeneous group of monogenic disorders with a series of symptoms including night blindness and progressive tunnel vision that eventually lead to blindness. The disease invariably involves death or dysfunction of rod photoreceptors and is caused by defects in several different molecular pathways. To date, almost 3,000 mutations in more than 56 disease-causing genes are known to be associated with nonsyndromic RP [1] , [2] . Despite the identification of an increasing number of disease-causing genes, a large proportion of patients with autosomal recessive RP (arRP) lack a genetic predisposition due to a mutation in one or more of the 36 known genes [1] , [2] . To gain further understanding of the genetics of arRP, we focused on patients who did not carry a defined genetic mutation in any of the previously reported genes. In one such kindred, the proband from a consanguineous family had severe early-onset RP. Here we perform targeted exome-capture sequencing of known genes to reveal the underlying genetic defect, but fail to identify any pathological mutations. Through whole-exome sequencing, we identify a homozygous missense mutation in a cationic amino acid transporter gene, SLC7A14 . Further, screening of this gene in 247 patients with arRP identifies an additional four unrelated patients with different mutations in the SLC7A14 gene. These mutations are absent from a database generated by exome sequencing of DNA from 300 in-house patients. Slc7a14 expression increases over the course of retinal development and remains abundant in the mature retina. Knockdown of slc7a14 in zebrafish causes a significant phenotype in the eye and an abnormal photomotor response. Furthermore, Slc7a14 -knockout mice are generated, and they demonstrated structural and functional abnormalities in the retina. Our findings identify a new disease gene underlying arRP and provide insight into SLC7A14 dysfunction in human retinal degeneration. Patients with early-onset RP In a first-cousin consanguineous family ( Fig. 1a ), a patient with sporadic RP had night blindness and a visual field defect, both of which first appeared during childhood. Visual acuity in both eyes had progressively decreased to hand motion only by the age of 35. Fundus photography and optical coherence tomography (OCT) revealed a typical intraretinal bone spicule pigmentation, large spots of retinal atrophy and overall thinning of the outer retinal layer, respectively ( Fig. 1b,c ). Electroretinogram (ERG) responses were extinguished ( Fig. 1d ). The patient’s parents and other relatives were unaffected. The severely affected structure and function of the retina support the clinical diagnosis of arRP. 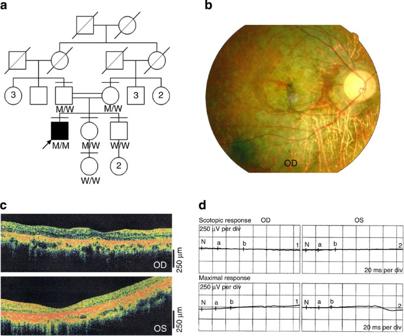Figure 1: Pedigree and clinical characteristics of a patient with arRP. (a) A simplified pedigree of the W60 family. The arrow pointing to the filled symbol indicates the index proband patient; the oblique lines indicate deceased subjects; the number in the box or circle indicates the number of unaffected siblings. M, mutation; W, wild-type. (b) Fundoscopy of the proband patient revealed extensive degeneration in both eyes. A representative image is shown. (c) OCT of the proband patient determined that the retinal thickness was significantly decreased. (d) The proband patient exhibited an extinguished response to an ERG. Figure 1: Pedigree and clinical characteristics of a patient with arRP. ( a ) A simplified pedigree of the W60 family. The arrow pointing to the filled symbol indicates the index proband patient; the oblique lines indicate deceased subjects; the number in the box or circle indicates the number of unaffected siblings. M, mutation; W, wild-type. ( b ) Fundoscopy of the proband patient revealed extensive degeneration in both eyes. A representative image is shown. ( c ) OCT of the proband patient determined that the retinal thickness was significantly decreased. ( d ) The proband patient exhibited an extinguished response to an ERG. Full size image Mutational screening of known RP-related genes To reveal the underlying genetic defect in this patient, we initially screened 144 genes that are known to be related to RP by using our established targeted exome-sequencing approach [3] . No pathological mutations were found in any of these known genes. Exome-sequencing detects a missense variant in SLC7A14 Because we did not identify mutations in any known RP-related genes, we performed whole-exome sequencing with the Nimblegen solid-phase array capture system and a Solexa HiSeq 2000 sequencer. The average sequencing depth and coverage of our analysis were 60.73% and 98.5%, respectively. The percentage of genes with >20 reads was 81.0%. A total of 20,652 small insertions and deletions (InDels) were identified by the GATK programme. Among them, 58 were selected through filtering with the 1k and HapMap databases. Further validation by Sanger sequencing and co-segregation analysis led to rejection of all of these InDels as the disease-causing mutation. Using the SOAPsnp programme [4] , we identified 10839 nonsynonymous variants. Among them, 3161 were selected by excluding those with a MAF >0.05. All SNPs were deposited in the HapMap 28 and 1000 Genomes Project databases. Computational prediction (Polyphen and SIFT) further excluded 2653 nonpathological SNPs and 508 variants were remained. As the affected probands in a consanguineous inbred family are likely to have two recessive disease alleles inherited from a common ancestor (that is, identical-by-descent), we focused on identifying homozygous mutations from our sequencing data. In this family, a total of 15 homozygous variants were found ( Supplementary Table 1 ). We performed the homozygosity analysis and our results demonstrated that the p.G330R change was inside a 3.1 MB homozygous region (chr3: 168802626-171969076). A total of 594 homozygous regions over 1 Mb were present and only six homozygous variants were inside the homozygous regions ( Table 1 ). Among them, two variants were excluded by co-segregation analysis in the family. The other three variants could also been excluded through gene expression pattern and reported diseases ( Table 1 ). 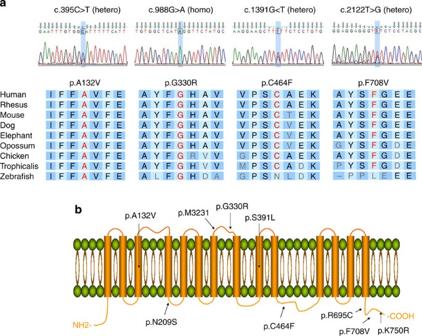Figure 2: Identification of mutations inSLC7A14in patients with arRP. (a) Sequence chromatograms illustrate the causal lesions that were identified in five unrelated patients with arRP. Each mutation leads to alteration of a highly conserved amino acid residue. (b) The identified mutations in the nontransmembrane (line) and transmembrane (column) domains of SLC7A14 predicted by SMART algorithms. As a result, the homozygosity analysis suggested a homozygous missense variant, c.988G>A (p.G330R), in exon 5 of the SLC7A14 gene (3q26.2) encoding the solute carrier family 7 (orphan transporter), member 14 as the possible genetic mutation underlying the disease ( Table 2 ). The mutation, which was validated by Sanger sequencing, is located in a codon for a highly conserved amino acid residue. In addition, it co-segregated with the disease in the pedigree ( Fig. 1a ). This finding suggests that it is a candidate mutation. Table 1 Six homozygous variants in the homozygous regions over 1 Mb. Full size table Table 2 SLC7A14 mutations identified in RP patients. Full size table Mutational screening in additional arRP cohorts To examine the mutation frequency of SLC7A14 in arRP, we screened a total of 247 unrelated patients with arRP. We identified four additional patients with arRP ( Supplementary Fig. 1 ) who had homozygous or compound heterozygous SLC7A14 mutations ( Table 2 ) co-segregated in each family ( Supplementary Fig. 2 ). These mutations were predicted to alterations of highly conserved amino acids between different species ( Fig. 2a and Supplementary Fig. 3 ). These patients were comprehensively screened by targeted exome sequencing of known RP-related genes [3] and no additional mutations were identified; the absence of additional mutations supports the hypothesis that mutations in SLC7A14 are the cause of RP. 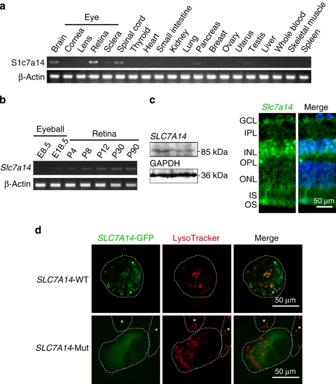Figure 3: Expression analysis and functional assay of theSLC7A14mutation. (a) High expression ofSLC7A14was observed in the retina, brain and spinal cord. (b)SLC7A14is expressed as early as stage E18.5 and expression increases during postnatal development of the retina. (c) Immunohistochemical analysis of the retina showed that SLC7A14 (green) is expressed in the photoreceptor layer. Rhodopsin (red) is expressed in the outer segment of rod photoreceptors. DAPI (blue) indicates DNA in the cells’ nuclei. Scale bar, 50 μm. (d)In vitroassay elucidated the mutation effect on Slc7a14 subcellular localization. Wild-type Slc7a14 is colocalized with LysoTracker, whereas the p.G330R mutant does not and exhibits a remarkable change with a diffuse distribution of the signal in the cytoplasm, demonstrating that the mutation affects protein subcellular localization. Scale bar, 50 μm. We also identified 12 patients with a single heterozygous variant ( Table 3 ), which computational analysis determined to be pathological and which were absent from an in-house whole-exome dataset that was obtained from 300 unrelated individuals. In one (W52-1) of these patients, a definitive mutation in RP1 gene (c.3469_3476del8bp) was identified ( Table 3 ). Another two probands had mutations successfully identified in the EYS and BEST1 genes ( Table 3 ). No copy-number variation of this gene was found by real-time PCR [5] in these patients with a heterozygous variant, consisting with the registered results in the Database of Genomic Variants (projects.tcag.ca/variation/). We speculated that these 12 additional probands carrying single heterozygous variants are not caused by the SLC7A14 mutation. With the exception of c.395C>T and c.1172C>T, all of the identified mutations were predicted to cause alterations of amino acid residues located in the extracellular or cytoplasmic domains ( Fig. 2b ). Notably, two mutations, c.988G>A and c.1391G>T, were found in 10 and 4 cases, respectively. Thus, these may be common mutations in the Chinese population. Collectively, these results serve as further evidence that mutations in SLC7A14 are pathogenic and indicate that the frequency of SLC7A14 mutations in Chinese patients with arRP is 2.0% (5 of 248 cases). Figure 2: Identification of mutations in SLC7A14 in patients with arRP. ( a ) Sequence chromatograms illustrate the causal lesions that were identified in five unrelated patients with arRP. Each mutation leads to alteration of a highly conserved amino acid residue. ( b ) The identified mutations in the nontransmembrane (line) and transmembrane (column) domains of SLC7A14 predicted by SMART algorithms. Full size image Table 3 Single heterozygous variants identified in arRP patients. Full size table Gene expression analysis The SLC7A14 gene contains seven coding exons (2316 nucleotides) and encodes a protein, cationic amino acid transporter, y+ system, with 771 amino acids. Its function remains largely unknown [6] . We investigated the expression profile in mouse tissues and found a high expression of SLC7A14 in both the brain and eye ( Fig. 3a and Supplementary Fig. 9 ). Furthermore, this gene is expressed as early as embryonic stage E18.5 and its expression increased during postnatal development of the mouse retina ( Fig. 3b and Supplementary Fig. 9 ). An immunohistological study of the mouse retinas detected specific Slc7a14 expression in the inner nuclear layer and photoreceptor layer ( Fig. 3c and Supplementary Fig. 9 ). This expression pattern is consistent with a potential disease-causing role of SLC7A14 mutations in RP. Figure 3: Expression analysis and functional assay of the SLC7A14 mutation. ( a ) High expression of SLC7A14 was observed in the retina, brain and spinal cord. ( b ) SLC7A14 is expressed as early as stage E18.5 and expression increases during postnatal development of the retina. ( c ) Immunohistochemical analysis of the retina showed that SLC7A14 (green) is expressed in the photoreceptor layer. Rhodopsin (red) is expressed in the outer segment of rod photoreceptors. DAPI (blue) indicates DNA in the cells’ nuclei. Scale bar, 50 μm. ( d ) In vitro assay elucidated the mutation effect on Slc7a14 subcellular localization. Wild-type Slc7a14 is colocalized with LysoTracker, whereas the p.G330R mutant does not and exhibits a remarkable change with a diffuse distribution of the signal in the cytoplasm, demonstrating that the mutation affects protein subcellular localization. Scale bar, 50 μm. Full size image The G330R mutation led to Slc7a14 dislocation To examine whether the identified missense mutation, p.G330R, affects Slc7a14 localization, we constructed a plasmid with the Slc7a14 missense mutation which was expressed in 293D cells. Immunocytochemistry revealed that wild-type Slc7a14 overlapped with the lysosome marker [6] , LysoTracker, whereas G330R-expressing cells showed a diffuse pattern of Slc7a14 expression throughout the cytoplasm ( Fig. 3d ). To test the arginine transport function, we performed an arginin transporting assay. Expression plasmid of either the wild-type or mutant Slc7a14 with G418 resistance was constructed and then transfected into photoreceptor cells (661W cell line). L-[3H]arginine transport assay show that photoreceptor cells with or without the G330R mutation in the Slc7a14 gene have the least concentration of transported L-[3H]arginine ( Supplementary Fig. 4 ) comparing with previous report [7] . A possible explanation might be that endogenous Slc7a14 remained in the G418-selected cells exert transport function. The results collectively suggested that the Slc7a14 missense mutation prevented the protein from localizing to the lysosome, where it would normally be degraded, which could contribute to the pathogenicity of the G330R mutation in the SLC7A14 gene. Knockdown of Slc7a14 in zebrafish To test our hypothesis that disruption of the slc7a14 gene can lead to visual dysfunction, we developed a zebrafish model of slc7a14 knockdown. Morpholino oligonucleotides (MOs) targeting the splice sites of the slc7a14 gene and a fluoresceinated standard control MO (Gene-Tools, LLC, Corvallis, OR) were microinjected into embryos at the one- to two-cell stage. The fluoresceins were observed after injection ( Supplementary Fig. 5a ) and RT–PCR verified the alteration in splicing ( Supplementary Figs 5b, 9 ). Injection of the slc7a14 -MO led to abnormal phenotypes in 46.9% of fish (total number of examined fish is 130). These phenotypes included smaller eyes (39.2%) and severe malformations (body disfigurement; 7.7%), whereas a normal phenotype was observed in 95.4% of fish ( n =108) injected with the control MO ( Supplementary Fig. 6 ). We did not observe significant retinal structural change in the 5dpf slc7a14 -MO zebrafish ( Supplementary Fig. 5c ). This finding suggests that knockdown of slc7a14 in zebrafish results in a significantly abnormal phenotype. Compared with the larvae that were injected with the control MO, larvae injected with the slc7a14-MO displayed an eye phenotype of significantly smaller eyes ( Fig. 4a,b ). To determine the effect of slc7a14 knockdown on visual function, we assessed the swimming response of 5dpf larvae to sudden light-to-dark transitions by using a previously established light-induced locomotor response [8] in conjunction with a ZebraBox behaviour monitoring station. The behavioural testing demonstrated that zebrafish larvae with reduced levels of slc7a14 exhibited an aberrant locomotor response during the light-ON phase ( Fig. 4c ). The aberrant behaviour was significantly different from the normal behaviour ( P <0.01, N =10, Dunnett test; Fig. 4d ). These findings strongly indicate that Slc7a14 has an important role in photoreceptor development and function and that its dysfunction can lead to visual impairment. 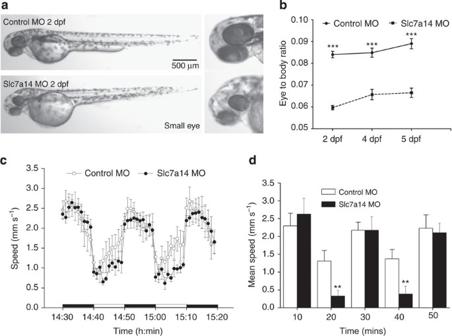Figure 4: Knockdown ofSLC7A14in zebrafish. (a) Injection of 1 nl of a 0.25 mM solution ofslc7a14-MO dramatically reduces eye size in zebrafish. (b) At 2dpf, 4dpf and 5dpf, the eye-to-body ratio of fish injected with theslc7a14-MO was significantly smaller than that of fish injected with the control MO.N=6, Dunnett test, ***P<0.001. (c) Light-induced locomotor response with sudden light-to-dark transitions demonstrated significant visual impairment in zebrafish injected with theslc7a14-MO.N=6 in each group. (d) Dunnett tests of the light-induced locomotor responses indicate that significant differences exist between the responses of fish with small eyes and those with normal eyes during the light-ON phase.N=10, Dunnett test, **P<0.01. Bars in the graph represent standard errors of the mean (s.e.m.). Figure 4: Knockdown of SLC7A14 in zebrafish. ( a ) Injection of 1 nl of a 0.25 mM solution of slc7a14 -MO dramatically reduces eye size in zebrafish. ( b ) At 2dpf, 4dpf and 5dpf, the eye-to-body ratio of fish injected with the slc7a14 -MO was significantly smaller than that of fish injected with the control MO. N =6, Dunnett test, *** P <0.001. ( c ) Light-induced locomotor response with sudden light-to-dark transitions demonstrated significant visual impairment in zebrafish injected with the slc7a14 -MO. N =6 in each group. ( d ) Dunnett tests of the light-induced locomotor responses indicate that significant differences exist between the responses of fish with small eyes and those with normal eyes during the light-ON phase. N =10, Dunnett test, ** P <0.01. Bars in the graph represent standard errors of the mean (s.e.m.). Full size image Generation and characterization of Slc7a14 -deficient mice The TALEN-mediated gene knockout approach was performed to induce targeted Slc7a14 gene disruption ( Fig. 5a ). TALEN repeats were designed to bind the exon 2 of the Slc7a14 gene. The repeats were fused with FokI restriction endonuclease [9] . After transfection of the TALEN constructs into the C6 cell line (No. TCR 1, SIBS Cell Bank, Shanghai, China), TALEN expression and activity were verified through western blot ( Supplementary Figs 7a, 9 ) and MSDase assay ( Supplementary Figs 7b, 9 ), respectively. In vitro -transcribed mRNA was microinjected into the pronuclei of C57BL/6 mice zygotes ( n =141). Among the 12 founder mice with Slc7a14 mutations, three mice were selected for further characterization because they had 10 bp-deletions in both alleles ( Supplementary Fig. 7c ), which introduced an earlier stop codon and led to Slc7a14 protein truncation. We found that the Slc7a14 -deficient mice were viable, fertile and did not show noticeable physical abnormalities ( Supplementary Fig. 7d ). 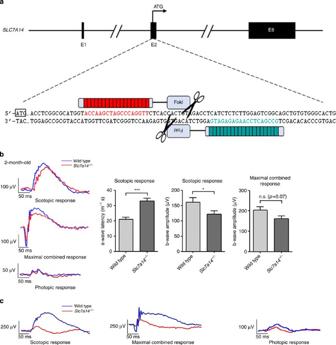Figure 5: Generation and characterization ofSlc7a14-knockout mice. (a) Schematic of theSlc7a14gene knockout strategy in mice. (b) ERG testing demonstrated a lower b-amplitude and a longer a-wave potential time in 2-month-oldSlc7a14−/−mice when compared with age-matched controls.N=3. Bar in the graph represents s.e.m. Student’st-test, *P<0.05; ***P<0.001. (c) The 6-month-old KO mice displayed severely decline of ERG responses. Figure 5: Generation and characterization of Slc7a14 -knockout mice. ( a ) Schematic of the Slc7a14 gene knockout strategy in mice. ( b ) ERG testing demonstrated a lower b-amplitude and a longer a-wave potential time in 2-month-old Slc7a14 −/− mice when compared with age-matched controls. N =3. Bar in the graph represents s.e.m. Student’s t -test, * P <0.05; *** P <0.001. ( c ) The 6-month-old KO mice displayed severely decline of ERG responses. Full size image A series of examinations, including electroretinography (ERG), OCT and retinal immunohistochemistry, were performed to test the visual function and to evaluate the retinal anatomy of the mice. ERG, an objective assessment of retinal function, showed that the ERG response was abnormal in the Slc7a14 -deficient mice aged 2-months ( Fig. 5b ) and 6-months ( Fig. 5c ). In addition, we use high-resolution OCT [10] , [11] and hematoxylin and eosin (HE) staining to investigate the retinal layer structure of the 2.5-month-old mice. The OCT results showed a trend of reduced thickness of the outer retina in the knockout mice ( Supplementary Fig. 8a ), whereas the result of HE staining also indicates a slightly thinner retinal layer in the 2.5-month-old KO mice ( Supplementary Fig. 8b ). Collectively, these data demonstrate that the ablation of Slc7a14 protein in mice leads to retinal degeneration. This degeneration recapitulates the disease phenotype in the arRP patients with SLC7A14 mutations. Pedigree-based genetic mapping has facilitated the discovery of many disease-causing genes. To date, 56 disease genes have been identified for nonsyndromic RP, including 23 for autosomal dominant RP (adRP), 36 for arRP (including six overlapping genes) and three for X-linked RP. Despite this progress, the genetic defect of more than half of the patients with arRP remains unknown [1] as it has been challengeable to screen all causative genes synchronously. Next-generation sequencing technologies employing high-throughput exomic screening have proven to be powerful tools for discovering new disease-related genes for RP and allied diseases [12] , [13] , [14] , [15] . Our study has further demonstrated the robustness of this approach: the use of exome sequencing allowed us to determine that SLC7A14 is a novel causative gene in a small RP pedigree. In this study, a homozygous mutation in the SLC7A14 gene (c.988G>A; MAF 0.005 in the Single Nucleotide Polymorphism database) was identified in the proband patient and the heterozygous mutation was confirmed in the patient’s parents. By screening additional families with arRP, we identified unique homozygous or compound heterozygous mutations in SLC7A14 in four unrelated patients. The SLC7A14 gene may contain hot spots for genetic mutation, because two mutations, c.988G>A and c.1391G>T, were frequently seen in the patients. Our results also demonstrate that SLC7A14 mutations are causative for arRP in 2.0% of the Chinese patients with this disease. Such a high percentage indicates that molecular diagnosis of patients with arRP should include mutational screening of SLC7A14 . The identification of SLC7A14 as an RP-causing gene raises an intriguing question as to how mutations in an orphan transporter gene that is expressed in the retina and throughout the central nervous system can lead to a retina-specific phenotype. This gene encodes an orphan transporter protein that has not been reported to be related to any other disease. Our study is the first to link SLC7A14 to retinal disease in humans. Previously, Jaenecke et al. [16] determined that SLC7A14 is localized to the lysosomal membrane and hypothesized that it might mediate transport of cationic amino acids across the lysosomal membrane. SLC7A14 was also shown to inhibit the ubiquitously expressed serine/threonine protein phosphatase-1 protein [17] , which is essential for normal development of the eye [18] . Thus, it is tempting to speculate that SLC7A14 mutations may lead to retinal degeneration via phosphatase-1 protein disinhibition. The exact role of SLC7A14 in photoreceptor cells remains to be elucidated and this topic warrants further investigation. In the present study, we generated the Slc7a14 -deficient mouse model, which would be very useful for elucidation of molecular mechanism as well as therapeutic intervention. To our knowledge, this is the first time that recurrent SLC7A14 mutations were identified in cases of arRP. Our results indicate that the mutation frequency of SLC7A14 in the population of Chinese patients with arRP is 2.0% (five independent cases among 248). Our functional characterization also supports the hypothesis that SLC7A14 is a new causative gene of arRP and provides new insights into the transporter-related disease mechanisms underlying RP. Therefore, mutational screening of SLC7A14 should be considered for patients with arRP to ensure proper molecular diagnosis. Subject recruitment and clinical examination This study was approved by the ethics committee of The Eye Hospital of the Wenzhou Medical University and informed consent was obtained from each participant. The protocol conformed to the tenets of the Declaration of Helsinki. A complete ophthalmic examination of each proband patient was carried out to clinically diagnose the disease and its severity. Targeted and whole-exome sequencing A total of 144 RP-targeted genes were captured and enriched as previously described [3] . In family W60, the proband patient, his unaffected sister and his parents were recruited to submit DNA for whole-exome sequencing. The DNA was first quantified with a Nanodrop 2000 (Thermal Fisher Scientific, DE, USA). A minimum of 3 μg of DNA was used to make the indexed Illumina libraries in accordance with the manufacturer’s protocol. The whole-exome region of the library was enriched by using the Exome Enrichment V5 Kit (Agilent Technologies, USA) in accordance with the protocol that was provided with the kit. Both the targeted and the whole-exome-enriched library were sequenced by using paired-end 100 bp reads and a HiSeq 2000 sequencer (Illumina, USA). Bioinformatics analysis For the quality control of raw data, we filtered low-quality reads by using the Trim Galore! programme. Then, the 3′ and 5′ adapters were trimmed by using the Cutadapt programme implemented in Trim Galore!. Only reads with a sequencing quality greater than 20 and a read length greater than 80 bp were retained. The filtered reads were aligned to the reference genome sequence by using the Burrows-Wheeler Aligner as a sorted binary. The Sequence Alignment/Map tools were used to remove duplications. The sequencing depth and coverage were calculated on the basis of the unique aligned reads. Single-nucleotide variants (SNVs) and InDels were identified by GATK. Standard GATK filters were applied to eliminate SNVs with strand bias, low quality for the depth of sequencing achieved, homopolymer runs and SNVs located near indels. The effects (for example, missense, nonsense or frameshift mutations) and classifications (for example, located in an exonic, intronic or intergenic region) of the variants were annotated across the genome by ANNOVAR. SLC7A14 amplification and genotyping The proband patient (W60-1) and the other subjects from families with arRP were selected to submit DNA for Sanger sequencing. Primers ( Supplementary Table 2 ) were designed to amplify all seven coding fragments and the intron–exon boundaries of the SLC7A14 gene. The PCR products were purified and sequenced on an ABI 3500 Genetic Analyser (Applied Biosystems, CA, USA). Reverse transcription-PCR Total RNA was extracted from murine (C57BL/6 strain) tissues including whole brain, retina, lens, sclera, cornea, spinal cord, thyroid, heart, small intestine, kidney, lung, pancreas, breast, testis, liver, blood, skeletal muscle, spleen (in males) and ovary and uterus (in females). Reverse-transcribed cDNAs were used as templates for PCR with SLC7A14 and β-actin primers. The products were then subjected to electrophoresis on a 1.5% agarose gel. Immunohistochemical analysis Paraformaldehyde-fixed eyes were embedded in paraffin and cut into 20-μm-thick sections. The sections were then used for HE staining and immunofluorescent analysis with rabbit anti-SLC7A14 (HPA045929, Sigma, USA) primary antibodies, and Alexa Fluor 488-, Alexa Fluor 568-, and Alexa Fluor 350-tagged secondary antibodies (Molecular Probes, USA). Images of the stained sections were obtained with a LSM710 laser-scanning confocal microscope (Zeiss, German). SLC7A14-GFP fusion constructs and expression in 293D Cells The SLC7A14 gene was amplified from human brain cDNA using hSLC7A14-full primers ( Supplementary Table 3 ) and inserted into pEGFP-N2 vector. Site-directed mutagenesis was performed by overlap PCR using the hSLC7A14-mut primer set ( Supplementary Table 3 ). 293D cells were cultured in regular conditioned medium and seeded on a coated glass slide (WHB) in 24-well plates. The pEGFP-N2-SLC7A14 recombinant vector was transfected into 293D cells using GenEscortII (Wisegen) according to manufacturer’s instruction. The cells were stained with 50 nM LysoTracker Red DND-99 (Invitrogen) and analysed by confocal laser-scanning microscopy (Zeiss). L-Arginine transport assay in 661W photoreceptor cells Restriction sites for BamH I and Kpn I were introduced in the SLC7A14 coding sequence as a silent mutation. The sequence of each oligonucleotide pair is presented in Supplementary Table 3 . The BamH I and Kpn I sites were used to create chimeric cDNAs between SLC7A14 and hCAT2. The chimeric cDNAs were subcloned into the pCDNA3.1(+) expression vector (Invitrogen) and were named as pcDNA3.1-hCAT2-SLC7A14-wt and pcDNA3.1-hCAT2-SLC7A14-mut, respectively. The 661W cells were transfected in six-well plates using Lipofectamine 2000 reagent (Invitrogen) according to the manufacturer’s protocol. Stably transfected cell clones were selected in medium containing 1 mg ml −1 G418. The selected 661W cells were plated at a density of 5 × 10 4 cells per well in 24-well cluster trays (Costar). Transport assays were performed using cluster trays as described by Gazzola and colleagues [19] . Cells were washed with 0.5 ml of Dulbecco’s phosphate-buffered saline (pH 7.4; Gibco), containing 0.9 mM CaCl 2 , 0.5 mM MgCl 2 , 2.7 mM KCl, 1.5 mM KH 2 PO 4 , 137 mM NaCl, 8.1 mM Na 2 HPO 4 and supplemented with 0.1% (w/v) glucose (PBSG). The 661W cells were incubated at 37 °C for 10 min in the medium supplemented with 100 μM unlabelled L-arginine and 5 μCi ml −1 L-[ 3 H]arginine (40-60 Ci mmol −1 ; American Radiolabeled Chemicals), followed by rapid decanting and shaking of the uptake medium into a receiving vessel. The 661W cells were immediately washed three times on ice with cold (4 °C) PBSG containing 10 mM unlabelled L-arginine with the cluster tray placed on ice. Cells were detergent-solubilized in 0.5% Nonidet P-40 and 0.1% SDS and finally the radioactivity of the extracts was quantified by liquid scintillation counting (ALOKA). Slc7a14 knockdown in zebrafish MOs were synthesized by Gene-Tools, LLC (Corvallis, OR, USA). The antisense sequence (25 bases) of the fluorescein-tagged MO targeting the splice site of the slc7a14 gene corresponds to that between the first intron and second exon of the coding region (5′-CAAGGCTGAGGACAGAATAAGATGA-3′). The sequence of the fluorescein-tagged standard control MO is as follows: 5′-CCTCTTACCTCAGTTACAATTTATA-3′. The MOs were diluted and approximately 1 nl of the 0.25 mM slc7a14 -MO and control MO solutions were microinjected into the embryos, which were at the one- to two-cell stage. To confirm the effectiveness of the MO injections and knockdown of Slc7a14 expression, fluorescence was assessed and RT–PCR analysis was conducted. Morphological analysis was carried out to measure the eye/body ratio as described previously [20] . In brief, the fish larvae were positioned for imaging. Body length was measured from the anterior tip to the posterior end of the body, whereas eye length was defined as the axial distance from anterior to the posterior part. Light-induced locomotor response To determine the effect of slc7a14 knockdown on the 5dpf larvae, we used the light-induced locomotor response test with sudden light-to-dark transitions. One larvae that had been injected with either the slc7a14 -MO or the control MO was placed in one well of a 24-well plate. The behaviour of the larvae was assessed in a ZebraBox behaviour monitoring station (ViewPoint Life Sciences, Montreal, Canada). The larva was allowed 20 min to adapt to visible light similar in intensity to the ambient overhead fluorescent lighting in the laboratory. After the adaptation period, the locomotor response, calculated as the average swimming speed per min, was recorded. The light cycle was 10 min of visible light followed by 10 min of darkness, repeated for 50 min. Each photomotor experiment was performed on a total of 6 fish for each group (fish injected with the slc7a14 -MO and those injected with the control MO). The Dunnett test was used for statistical analysis of the data. Generation of TALEN-mediated Slc7a14 -knockout mice TALEN repeats were designed to bind the exon 2 of Slc7a14 gene and fused to a FokI nuclease domain ( Fig. 5a ). Slc7a14 -specific TALEN plasmids were generated and transfected into C6 cells. Western blotting analysis was performed to confirm its expression and MSDase assay was carried out to examine the TALEN activity. In vitro -transcribed Slc7a14-TALEN mRNAs were prepared and microinjected into fertilized eggs of C57BL/6 mice, which were transferred to pseudopregnant females. All mice were maintained in the specific pathogen-free facility. Newborn pups were genotyped by PCR using tail-derived DNAs. Full-field ERGs ERGs of Slc7a14 -deficient mice and age-matched wild-type mice were recorded as previously described [21] . Both the scotopic and photopic ERGs were recorded with a well-established Ganzfeld dome stimulating and recording system. In brief, mice were dark-adapted, anesthetized. Pupils were dilated and an Ag/AgCl wire loop electrode was placed over the cornea. Scotopic ERG was recorded at 0.4 log cd-s m −2 intensity with a 30-sec inter-stimulus interval, and photopic ERG was measured at 1.4 log cd-s m −2 in the presence of 30 cd m −2 background light after 10 min of light adaptation. High-resolution OCT A customized high-resolution OCT instrument was used to image the mouse retina [11] , [12] . After anesthetization of the mice, the pupils were fully dilated with 0.2% tropicamide. The mice were placed on a custom built stage to facilitate imaging of the optic nerve head. Outer nuclear layer, inner segment and outer segment were segmented by using a well-established algorithm [22] , [23] . Accession codes: Whole-exome sequence data for the W60 family has been deposited in GenBank Sequence Read Archive (SRA) under the accession code SRP038008 . How to cite this article: Jin, Z.-B. et al. SLC7A14 linked to autosomal recessive retinitis pigmentosa. Nat. Commun. 5:3517 doi: 10.1038/ncomms4517 (2014).